Extraordinary carrier multiplication gated by a picosecond electric field pulse The study of carrier multiplication has become an essential part of many-body physics and materials science as this multiplication directly affects nonlinear transport phenomena, and has a key role in designing efficient solar cells and electroluminescent emitters and highly sensitive photon detectors. Here we show that a 1-MVcm −1 electric field of a terahertz pulse, unlike a DC bias, can generate a substantial number of electron–hole pairs, forming excitons that emit near-infrared luminescence. The bright luminescence associated with carrier multiplication suggests that carriers coherently driven by a strong electric field can efficiently gain enough kinetic energy to induce a series of impact ionizations that can increase the number of carriers by about three orders of magnitude on the picosecond time scale. Impact ionization originates from the Coulomb interaction between carriers and is essentially the reverse of the Auger recombination process [1] . In this process, a highly energetic conduction-band electron ( e 11 ) colliding with a valence-band electron gives two conduction electrons ( e 12 + e 22 ) and a hole ( h 21 ). The electron e 11 gains energy in the strong electric field, and this energy gain implies that carriers driven without being affected by incoherent phonon scattering efficiently acquire enough kinetic energy to trigger a series of impact ionizations, that is, carrier multiplication [2] , [3] . This multiplication process has an important role in the efficient working of photovoltaic nanomaterials [4] , [5] , [6] , [7] , electroluminescent emitters [8] , [9] and highly sensitive photon detectors used in optical quantum information applications [10] . However, despite the fact that carrier-initiated impact ionization in a strong electric field critically affects non-equilibrium quantum transport phenomena [11] , [12] , [13] , [14] , the elementary process of carrier scattering relevant to ballistic transport has yet to be clarified. Intense terahertz (THz) pulse sources have the potential to provide significant insights into ultra-fast carrier multiplication through purely optical methods, because a THz pulse has a high electric-field amplitude (>0.1 MVcm −1 ) and lasts a picosecond [15] , [16] , [17] . It has been shown that electrons in the conduction band of GaAs undergo ballistic motion without incoherent longitudinal optical (LO) phonon scattering for periods on time scales of hundreds of femtoseconds (2π ω LO − 1 =115 fs, where ω LO is the angular frequency of the LO phonon) [18] . Carriers accelerated ballistically on ultra-short time scales can therefore be expected to gain kinetic energy more efficiently and thereby trigger carrier multiplication. However, insufficiently strong THz pulses generate few carriers [19] , and various additional phenomena observed by THz and optical absorption measurements—such as phonon absorption [20] , intervalley scattering [21] and exciton dissociations [22] , [23] —obscure the carrier multiplication. In this article, we highlight the extraordinarily efficient carrier multiplication in the typical semiconductor GaAs when it is subjected to a THz pulse of a strong electric field. We demonstrate for the first time that the electric field of a THz pulse, unlike a DC bias, can generate a substantial number of excitons that emit near-infrared luminescence without any help from band-to-band photoexcitation. Our results imply that the carriers coherently driven by a strong electric field can efficiently gain enough kinetic energy to induce a series of impact ionizations that can increase the number of carriers by about three orders of magnitude on the picosecond time scale. Carrier multiplication with THz pulse excitation We developed an experimental scheme for studying carrier multiplication in nominally undoped GaAs quantum wells (QWs) with intense THz pulses ( Fig. 1a , Methods). Carrier multiplication was induced by irradiating the QW sample with a nearly half-cycle THz pulse lasting 1 ps and having a maximum peak electric field amplitude of 1.05 MVcm −1 (Methods) [24] . The THz pulses were focused onto a GaAs QW sample that was mounted on the cold finger of a helium-flow cryostat. The electric field polarization was perpendicular to the stacking direction and along the (100) direction of the sample. As the thickness of the QWs ( L =6 μm) is sufficiently thin compared with the centre wavelength of THz pulse (~300 μm; Fig. 1b ), the constructive interference inside the sample modifies the strength and shape of the incident THz pulse (Methods). 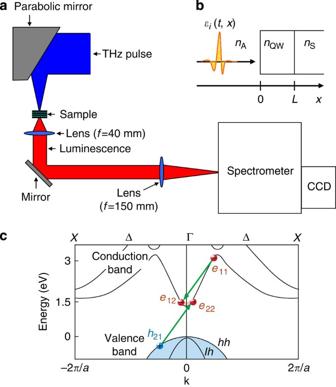Figure 1: Measurement of THz pulse induced luminescence and impact ionization process. (a) Generated THz pulses are focused onto the GaAs QWs sample, and the luminescence is detected by a CCD camera after it has passed through a spectrometer. (b) The geometry of the sample interfaces with air (nA=1), QWs (nQW=3.5) and a quartz substrate (nS=2.1). We assume here that the QWs with thickness (L=6 μm) on the quartz substrate has a homogeneous refractive index (nQW=3.5) represented by the average of the refractive indices of the wells (nw=3.6) and barriers (nb=3.4).ɛi(t,x) is incident THz electric field from the air. (c) Electron-initiated impact ionization transitions in the schematic GaAs band structure for momentum in the Δ direction. The lattice constantaof GaAs is 5.6 Å, and ±2π/acorresponds to ±1.1×1010m−1. The diagram shows electrons and hole positions before and after the transition at the threshold. Figure 1: Measurement of THz pulse induced luminescence and impact ionization process. ( a ) Generated THz pulses are focused onto the GaAs QWs sample, and the luminescence is detected by a CCD camera after it has passed through a spectrometer. ( b ) The geometry of the sample interfaces with air ( n A =1), QWs ( n QW =3.5) and a quartz substrate ( n S =2.1). We assume here that the QWs with thickness ( L =6 μm) on the quartz substrate has a homogeneous refractive index ( n QW =3.5) represented by the average of the refractive indices of the wells ( n w =3.6) and barriers ( n b =3.4). ɛ i ( t , x ) is incident THz electric field from the air. ( c ) Electron-initiated impact ionization transitions in the schematic GaAs band structure for momentum in the Δ direction. The lattice constant a of GaAs is 5.6 Å, and ±2 π / a corresponds to ±1.1×10 10 m −1 . The diagram shows electrons and hole positions before and after the transition at the threshold. Full size image The field ionization due to the THz pulse caused electrons from residual impurity donors to be accelerated along the Δ line around the Brillouin zone centre (Γ point) in momentum space as shown in Figure 1c (see the Methods section for a description of the field ionization) [25] . When the electric field reached a certain strength, the electrons acquired enough energy to induce several impact ionizations and produce substantial numbers of electron–hole ( e–h ) pairs that go on to form excitons around the Γ point. The impulsive electric field of the pulse allowed the unbound e–h pairs to form excitons that decayed radiatively because the electric field that would otherwise ionize the exciton was absent just after the pairs were generated [22] , [23] , [26] . The luminescence from the excitons was detected by a liquid-nitrogen-cooled charge-coupled device (CCD) camera ( Fig. 1a ). 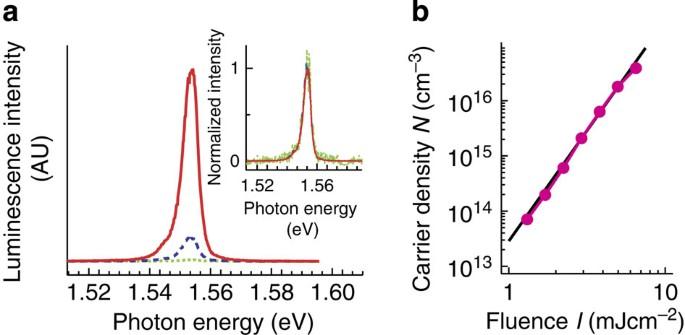Figure 2: Luminescence induced by intense THz pulses. (a) Spectra of luminescence excited at 10 K by THz pulses with peak electric field amplitudes of 0.54 MVcm−1(green dotted line), 0.70 MVcm−1(blue dashed line) and 1.05 MVcm−1(red solid line). Inset: normalized luminescence spectrum excited with the different electric field strengths. (b) THz pulse excitation intensity dependence of peak luminescence intensity (magenta closed circles). The eye guide (black solid line) corresponds to a fourth-power-law intensity dependence. Excitation intensity dependence Figure 2a clearly shows that THz pulses with different field strengths induce near-infrared luminescence centred around 1.55 eV from QWs at 10 K, even though the central photon energy of the pulse (~4 meV) is about 390 times lower than the luminescence photon energy [24] , and the luminescence intensity drastically decreases as the electric field ɛ decreases. As luminescence is proportional to the created e–h pair density [27] , the generated carrier density N can be estimated by comparing the luminescence measurement with optical pulse excitation measurements (Methods). As shown in Figure 2b , the carrier density N plotted as a function of THz pulse fluence I is extremely nonlinear and roughly proportional to I 4 ( ɛ 8 ). The minimum and maximum fluences correspond to electric fields of 0.47 and 1.05 MVcm −1 , and the carrier density increases over this range by about three orders of magnitude. Moreover, the shape of the emission spectra does not have any field dependence (inset of Fig. 2a ), which suggests that high-density excitation phenomena do not occur at these excitation intensity energies [28] . Figure 2: Luminescence induced by intense THz pulses. ( a ) Spectra of luminescence excited at 10 K by THz pulses with peak electric field amplitudes of 0.54 MVcm −1 (green dotted line), 0.70 MVcm −1 (blue dashed line) and 1.05 MVcm −1 (red solid line). Inset: normalized luminescence spectrum excited with the different electric field strengths. ( b ) THz pulse excitation intensity dependence of peak luminescence intensity (magenta closed circles). The eye guide (black solid line) corresponds to a fourth-power-law intensity dependence. Full size image Origin of luminescence We attempted to identify the origin of the observed luminescence by comparing the luminescences induced by a 1.05 MVcm −1 THz pulse and by a 3.18-eV optical pulse. 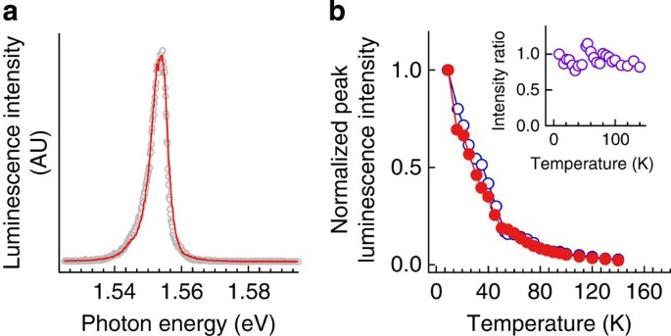Figure 3: Comparison of luminescence obtained by THz and optical pulse excitations. (a) Spectra of luminescence at 10 K excited by a 1.05 MVcm−1THz pulse (red solid line) and optical pulse with centre photon energy of 3.18 eV (grey open circles) (fluence absorbed by the sample is ~6 μJcm−2). (b) Temperature dependence of peak luminescence intensities excited by THz (red closed circles) and optical pulses (blue open circles). Inset: temperature dependence of intensity ratios as calculated by dividing the peak luminescence intensity due to a THz pulse by that due to the optical pulse (purple open circles). As shown in Figure 3a , the spectral shapes are almost the same, and the peak photon energies are near the heavy-hole ( hh ) exciton absorption peak. The luminescence induced by the THz pulse can therefore be inferred to be from radiative recombination of hh excitons. Figure 3b shows the temperature dependence of peak luminescence intensities obtained from the THz and optical pulse excitations. The temperature dependences are very similar, suggesting that these two kinds of pulses induce similar non-radiative decay processes of e–h pairs that contribute in almost the same way to their recombination processes. The ratio plotted in the inset of Figure 3b shows almost no temperature dependence, and this means that the exciton generation processes driven by THz pulses and optical pulses have similar temperature dependences. In contrast to the similar temperature dependences, the extremely nonlinear enhancement of luminescence intensity as a function of THz field strength nevertheless indicates that the e–h pair creation mechanism due to THz-pulse irradiation is completely different from the one due to photoexcitation. Figure 3: Comparison of luminescence obtained by THz and optical pulse excitations. ( a ) Spectra of luminescence at 10 K excited by a 1.05 MVcm −1 THz pulse (red solid line) and optical pulse with centre photon energy of 3.18 eV (grey open circles) (fluence absorbed by the sample is ~6 μJcm −2 ). ( b ) Temperature dependence of peak luminescence intensities excited by THz (red closed circles) and optical pulses (blue open circles). Inset: temperature dependence of intensity ratios as calculated by dividing the peak luminescence intensity due to a THz pulse by that due to the optical pulse (purple open circles). Full size image We attribute the generation of substantial numbers of carriers to highly efficient carrier multiplication triggered by impact ionizations rather than to Zener tunnelling. Note that we can exclude Zener tunnelling as a cause because the tunnelling occurring under a 1 MVcm −1 DC electric field lasting 1 ps can account for only a small amount of the e–h pairs (10 11 cm −3 ) [29] , far too small to explain the observation ( Fig. 2b ). In the impact ionization process [1] , an electron in the conduction band ( e 11 ), with kinetic energy gained from the electric field, creates an electron ( e 12 ) plus an e–h pair ( e 22 + h 21 ) ( Fig. 1c ): In accordance with energy and momentum conservation, this process is possible only if the electron has a threshold kinetic energy E th higher than the band gap E g of 1.52 eV. Here, E th = E g (2 m e + m hh )/( m e + m hh )=1.7 eV [30] , where m e (=0.067 m 0 ) and m hh (=0.5 m 0 ) are the effective masses of the electron and heavy hole, respectively. 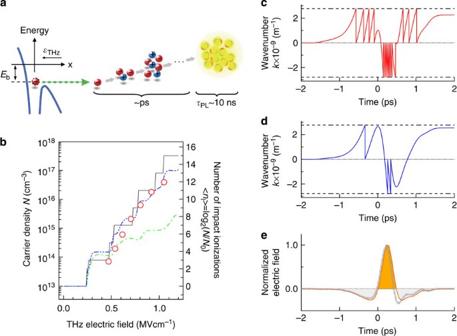Figure 4: Comparison of experimentally and theoretically obtained carrier densities. (a) The sketch visualizes the distortion in the Coulomb potential of donors, causing the potential to widen and free electrons to be released, and subsequent evolution of unbounde-hgas generated by a series of impact ionizations into a pure population of excitons emitting luminescence. (b) Electric field dependences of carrier density obtained in the experiment (red open circle) and calculations using equation (2) for three different impact ionization rates γIcal; one is infinity (grey solid line), and the others are derived from equation (3) withC=C0=870 ps−1eV−2(green one-dot-dashed line) andC=5C0(blue two-dot-dashed line). We assumedN0=1013cm−3. For the experimental (red open circles) and calculated data (grey solid line), the carrier densityNis plotted together with the corresponding 〈nI〉. Panels (c) and (d) show the electron wavenumberk(t) calculated by using equation (2) forɛ=1.05 and 0.47 MVcm−1, respectively. Dashed lines indicate the wavenumbers in the range of ±2.77×109m−1, where the electron energy corresponds to the threshold energyEthof 1.7 eV determined from the dispersion of the GaAs band structure. (e) Normalized electric field of the temporal profile of the incident THz pulse (grey dotted line) and of THz pulse with multiple reflections inside the sample (orange solid line). As shown in the sketch of Figure 4a , if an electron released from an impurity donor can be accelerated to the threshold kinetic energy, it can create an e–h pair ( Fig. 1c ). Subsequently, both the electron that lost energy to create the e–h pair and the created e–h pair could, in turn, gain energy from the field. This process can continue as long as the electric field of the THz pulse remains sufficiently strong, and so, comparably few impact ionization events can nevertheless produce numerous e–h pairs. Figure 4: Comparison of experimentally and theoretically obtained carrier densities. ( a ) The sketch visualizes the distortion in the Coulomb potential of donors, causing the potential to widen and free electrons to be released, and subsequent evolution of unbound e-h gas generated by a series of impact ionizations into a pure population of excitons emitting luminescence. ( b ) Electric field dependences of carrier density obtained in the experiment (red open circle) and calculations using equation (2) for three different impact ionization rates γ I cal ; one is infinity (grey solid line), and the others are derived from equation (3) with C = C 0 =870 ps −1 eV −2 (green one-dot-dashed line) and C =5 C 0 (blue two-dot-dashed line). We assumed N 0 =10 13 cm −3 . For the experimental (red open circles) and calculated data (grey solid line), the carrier density N is plotted together with the corresponding 〈 n I 〉. Panels ( c ) and ( d ) show the electron wavenumber k ( t ) calculated by using equation (2) for ɛ =1.05 and 0.47 MVcm −1 , respectively. Dashed lines indicate the wavenumbers in the range of ±2.77×10 9 m −1 , where the electron energy corresponds to the threshold energy E th of 1.7 eV determined from the dispersion of the GaAs band structure. ( e ) Normalized electric field of the temporal profile of the incident THz pulse (grey dotted line) and of THz pulse with multiple reflections inside the sample (orange solid line). Full size image This intuitive consideration of the multiplication dynamics leads to a prediction that can be compared with experimental observation. As can be seen in equation (1), an electron-initiated impact ionization event doubles the number of electrons. That is, given an initial electron density N 0 , the electron and hole densities after 〈 n I 〉 impact ionization events are, respectively, N 0 × 2 〈 n I 〉 and N 0 × ( 2 〈 n I 〉 - 1 ) . We can neglect the contribution of the generated heavy holes because their large effective mass would increase the threshold energy E th to 2.9 eV. Thus, the increase in impact ionizations 〈Δ n I 〉 that is due to changing the electric field from ɛ min =0.47 to ɛ max =1.05 MVcm −1 can be evaluated from the results to be log 2 ( N ( ɛ max )/ N ( ɛ min ))~9 (red open circles in Fig. 4b ). That is, at least nine impact ionizations on average occur within the 1-ps duration of the THz pulse. Hence, the impact ionization rate γ I for the maximum peak electric field is ~9/1×10 −12 s–10 13 s −1 . The experimentally obtained impact ionization rate γ I can be quantitatively compared with a simple theoretical prediction, whereby the motion of an electron in an electric field follows the dispersion of the band structure in momentum space. Here, we take the number of impact ionization events 〈 n I ( ɛ )〉 to be the number of times the average kinetic energy of the electrons reaches the E th of 1.7 eV; the GaAs dispersion relation provides this E th at a wavenumber k of ±2.77×10 9 m −1 (ref. 25 ). The change in electron wavenumber k ( t ) is solely determined by the electric field ɛ ( t ) acting on the electrons, because of the negligible influence of phonon scattering processes during periods of hundreds of femtoseconds [19] : where e is the electron charge and is Planck's constant. Here, we used the electric field of a THz pulse with multiple reflections inside the sample (Methods). The change in electron wavenumber k ( t ) during the THz pulse is calculated under the assumption that the electrons lose all their kinetic energy when they reach the average wavenumber ±2.77×10 9 m −1 , that is, an infinite impact ionization rate γ I cal of electrons ( Fig. 4c–e ). Accordingly, the e-h densities N ( ɛ ) after the 〈 n I ( ɛ )〉 impact ionization events can be estimated to be N 0 × 2 〈 n I 〉 (grey solid line in Fig. 4b ). The theoretical increase in number 〈Δ n I 〉 from ɛ min =0.47 to ɛ max =1.05 MVcm −1 is 〈 n I ( ɛ max ) 〉−〈 n I ( ɛ min )〉=12, and this estimate would also be subject to an uncertainty of around ±30%, owing mainly to the error in measuring the strength of the THz electric field. Hence, we can say it is close to the experimentally obtained 〈Δ n I 〉, and it confirms the validity of the experimentally derived γ I of ~10 13 s −1 . This high-impact ionization rate means that there are too few phonon interactions to prevent carriers from being driven coherently and multiplied efficiently during intervals of hundreds of femtoseconds. This conclusion is consistent with the temperature independence of the luminescence intensity ratio (see the inset of Fig. 3b ). If phonon scattering were a significant process on the sub-picosecond time scale, the efficiency of carrier generation due to THz pulse irradiation would be lower and the ratio would decrease with increasing temperature and phonon population. The assumption of an infinite γ I cal is reasonable only if the impact ionization time τ I =(γ I cal ) −1 is sufficiently short compared with the time τ a for the electron energy to reach E th from zero. The similar values of 〈Δ n I 〉 between the experiment (~9 times) and calculation (~12 times) suggest that τ I is sufficiently shorter than τ a . If the values were otherwise, the experimentally derived 〈 n I 〉 would be suppressed and the carrier multiplication could not occur so as to induce a 1000-fold increase in carrier density. We also theoretically analysed the observed carrier density with a finite impact ionization rate γ I cal , which is modelled according to the well-established Keldysh formula [32] : The corresponding values for electrons are taken from Fischetti and Laux [31] : C = C 0 =870 ps −1 eV −2 and E th =1.7 eV. As shown in Figure 4b , when we use a value of C =5 C 0 in equation (3), the calculation (blue two-dot-dashed line) reproduces the experimentally observed carrier density and is close to the curve calculated under the assumption of infinite γ I cal (grey solid line). Here, γ I cal =2.5×10 14 s −1 can be derived by using equation (3) with C =5 C 0 and E =1.94 eV at the maximum first-conduction-band energy between Γ and X points. The value γ I (~10 13 s −1 ) obtained experimentally is almost ten times smaller than the calculated γ I cal . The finite time for electrons to accelerate to E th can be the reason for the lower experimental value. The observed saturation behaviour at stronger electric fields in Figure 4b can be qualitatively understood to be from an enhancement in Coulomb scattering among the generated carriers. 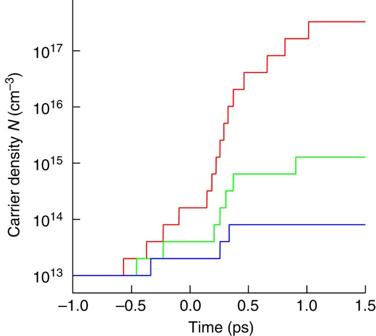Figure 5: Results of model calculation. (a) Calculated carrier densityN(t) as a function of time for different electric field strengths, which can be calculated by usingN0×2〈nI〉and the time development of impact ionization events 〈nI〉 during the THz pulse; 0.47 MVcm−1(blue solid line), 0.70 MVcm−1(green solid line) and 1.05 MVcm−1(red solid line). Figure 5 plots the carrier density in the QWs sample as a function of time, which can be calculated by using N 0 × 2 〈 n I 〉 and the time development of impact ionization events 〈 n I 〉 during the THz pulse ( Fig. 4c–e ). Under strong electric fields, the substantial numbers of e–h pairs generated at the earlier stage of multiplication may undergo a significant amount of e–h scattering. The scattering decelerates the electrons and reduces their ability to gain kinetic energy. Moreover, e - e scattering could lead to a redistribution of energy within the electron system, which may in turn reduce the average kinetic energy of a given carrier below the threshold and suppress the impact ionization events. Eventually, unbound e–h pairs generated with an energy conversion efficiency of ~5×10 −4 (Methods) may form excitons that have a relaxation time τ PL of several nanoseconds ( τ PL as determined by the radiative and non-radiative relaxation times; see Fig. 4a ). Figure 5: Results of model calculation. ( a ) Calculated carrier density N ( t ) as a function of time for different electric field strengths, which can be calculated by using N 0 × 2 〈 n I 〉 and the time development of impact ionization events 〈 n I 〉 during the THz pulse; 0.47 MVcm −1 (blue solid line), 0.70 MVcm −1 (green solid line) and 1.05 MVcm −1 (red solid line). Full size image In conclusion, we demonstrated extraordinarily high carrier multiplication in the typical semiconductor GaAs when it is subjected to a THz pulse of a strong electric field; the number of carriers increased by about three orders of magnitude. The carrier multiplication increase that occurs with an increase in the THz electric field was in agreement with phenomenological theory based on an impact ionization model including electron motion in k -space with a pristine band structure. In the future, a full quantum kinetic theory treatment of carrier dynamics in a band structure modified by an intense THz electric field should be performed to reveal the microscopic origin of the carrier multiplication [32] . Moreover, an experiment with a time-delayed probe pulse would allow for the carrier multiplication dynamics to be directly probed. Our findings of efficient ultra-fast carrier multiplication bode well for future applications in ultra-high-speed devices such as high-quantum-efficiency THz-biased avalanche photodiodes that have femtosecond resolution and are sensitive to a single photon, and they may also be exploited in the development of efficient electroluminescent and photovoltaic nanoscale devices. Samples A sample of nominally undoped GaAs/Al 0.3 Ga 0.7 As QWs was grown by molecular beam epitaxy on a (100)-GaAs substrate. It consisted of 272 periods of GaAs QWs (11.9 nm) separated from each other by Al 0.3 Ga 0.7 As barriers (10 nm). We removed the GaAs substrate by wet etching and placed the QWs film on a Z-cut quartz substrate ( Fig. 1b ). The dominant donor impurities were sulphur from an arsenide source. The static electric field ɛ ion necessary to ionize the sulphur donor is estimated as ɛ ion = E b / ea B ~4 kVcm −1 , where e is the charge of the electron and E b and a B are the binding energy and Bohr radius of the impurity donor in bulk GaAs, respectively. The E b given by the literature is ~6 meV, and a B (= ɛ 0 a 0 m 0 / m * ) is estimated to be ~10 nm, where ɛ 0 =12.4 and m * =0.067 m 0 are the dielectric constant and effective mass of an electron in bulk GaAs, respectively, and a 0 is the Bohr radius in the hydrogen atom [33] . This ionizing field is much lower than the minimum peak field of 0.47 MVcm −1 to see the luminescence. Consequently with this set up, the donors are completely ionized during the rise time of each THz pulse, and the released electrons trigger the carrier multiplication process ( Fig. 4a ). Measurements High-electric-field THz pulses were generated by optical rectification of femtosecond laser pulses in LiNbO 3 by using the tilted-pump-pulse-front scheme [15] , [16] , [17] , [24] . For the pump source, we used an amplified Ti:sapphire laser that provided a pulse energy of 4 mJ, a full width at half-maximum intensity of 85 fs, a central wavelength of 780 nm and a repetition rate of 1 kHz. The optical pulses from the oscillator with a repetition rate of 80 MHz synchronized with the amplified pulses were used for electro-optic sampling of THz pulses at the sample position [24] . The THz pulse energy measured by a pyroelectric detector (MicroTech Instruments, Inc.) was 2.3 μJ at an electric field of 1.05 MVcm −1 . The generated luminescence was analysed with a spectrometer with a resolution of about 1 meV and detected by a liquid-nitrogen-cooled CCD camera. To prevent stray near-infrared pulse laser light from entering the CCD camera, we put a black polypropylene sheet whose Fresnel coefficient for transmission in the THz frequency region was 0.87 in front of the cryostat window. To change the THz pump fluence, we put black polypropylene sheets in the THz-beam path. Electric field of the THz pulse inside the sample Figure 1b shows the geometry of the sample interfaces with air ( n A =1) and the quartz substrate ( n S =2.1). We assume here that the QWs has a homogeneous refractive index n QW that is the average of the refractive indices of the wells ( n w =3.6) and barriers ( n b =3.4), that is, 3.5. The electric field ɛ ( t , x ) inside the QWs in which multiple reflections take place can be written as follows: where ɛ i ( t , x ) is incident THz electric field from the air, N is the number of round trips, c is the speed of light, [ttilde]=2/( n QW +1) is the Fresnel transmittance between the air and sample, [ttilde] 1 =( n QW −1)/( n QW +1) is the Fresnel reflectance at the air and sample interface, [ttilde] 2 =( n QW − n S )/( n QW + n S ) is the Fresnel reflectance at the sample and substrate interface and τ 0 = n QW L /c is the phase shift. L is the thickness of the QWs. Consequently, the ratio of the maximum values of the positive lobe between the 6-μm thick and an infinitely thick QWs increases to 1.2. The maximum peak electric field inside the sample is estimated to be 0.55 MVcm −1 in the case of a 1.05 MVcm −1 electric field incidence. Estimation of carrier density The carrier density N generated by a 1.05 MVcm −1 THz pulse can be estimated by the following equation, where C THz is the total number of carriers and d w (=3.2 μm) is the length of the sample's GaAs wells alone (excluding the AlGaAs barriers). The effective diameter of the excited spot area a eff (~100 μm) is obtained by dividing the spot diameter in the electric field a in (~300 μm) by a factor of , as the generated carrier density roughly follows an 8th power law of the incident electric field ( Fig. 2b ). We obtained the same PL intensity with a THz pulse with a peak field value of ɛ max as with an optical pulse with a photon energy p of 3.18 eV, a spot diameter a opt of ~100 μm and absorbed fluence F of 6 μJcm −2 . The carrier numbers were about the same because the spot diameters of a eff and a opt were almost the same value (~100 μm). Accordingly, , where e =1.6×10 −19 eV −1 J. (The uncertainties of the carrier densities N are typically ±50%, owing mainly to the errors in the measurement of the optical excitation fluence and spot diameter of the THz pulse.) Energy conversion efficiency The energy conversion efficiency Q from the THz pulse energy W IN THz absorbed in the sample with respect to the impact ionization process W ii can be estimated from the generated carrier density. Part of the absorbed energy of the incident THz pulse goes into the impact ionization process; the other parts go into free carrier absorption and the transmitted THz pulse. The efficiency Q is defined as where E th =1.7 eV is the threshold energy of impact ionization. As the absorbed THz pulse energy W IN THz is almost 1 μJ, the conversion energy efficiency Q is estimated to be ~5×10 −4 . H.H. conducted the experiments and wrote the paper. H.H. and K.S. performed the measurements and analysed the data. H.H., K.S., M.S. and S.T. modelled the data. Y.K. designed and fabricated the sample. H.H. and K.T. initiated and provided management oversight for this project. All authors contributed to discussions and the final manuscript. How to cite this article: Hirori, H. et al . Extraordinary carrier multiplication gated by a picosecond electric field pulse. Nat. Commun. 2:594 doi: 10.1038/ncomms1598 (2011).